Atomic-scale mechanisms of ferroelastic domain-wall-mediated ferroelectric switching Polarization switching in ferroelectric thin films occurs via nucleation and growth of 180° domains through a highly inhomogeneous process in which the kinetics are largely controlled by defects, interfaces and pre-existing domain walls. Here we present the first real-time, atomic-scale observations and phase-field simulations of domain switching dominated by pre-existing, but immobile, ferroelastic domains in Pb(Zr 0.2 Ti 0.8 )O 3 thin films. Our observations reveal a novel hindering effect, which occurs via the formation of a transient layer with a thickness of several unit cells at an otherwise charged interface between a ferroelastic domain and a switched domain. This transient layer possesses a low-magnitude polarization, with a dipole glass structure, resembling the dead layer. The present study provides an atomic level explanation of the hindering of ferroelectric domain motion by ferroelastic domains. Hindering can be overcome either by applying a higher bias or by removing the as-grown ferroelastic domains in fabricated nanostructures. Ferroelectric thin films usually possess polydomain structures determined by electromechanical boundary conditions. For example, ferroelastic twinning structures with polarization rotations of 71° or 109° in rhombohedral perovskites (for example, BiFeO 3 ) or of 90° in tetragonal perovskites (for example, PbZr 0.2 Ti 0.8 O 3 (PZT)) provide an energetically favourable means of reducing the strain energy in epitaxial thin films. Many properties of ferroelectric thin films are closely correlated to the structure and dynamic behaviour of domains, and thus can be manipulated by domain engineering. For example, the piezoelectric response in epitaxial PZT thin films is particularly sensitive to embedded ferroelastic domains and can be dramatically enhanced by manipulating the domain structure to either remove these domains or increase their mobility [1] . Above a critical film thickness of about 100 nm in PZT [1] , [2] , stress-relieving ferroelastic domains generally form a dense square network of crossing domains, which, in epitaxial thin films, are usually nearly immobile because of the strong coupling between charge and strain in the system. Given the high density and poor mobility of such ferroelastic domains in epitaxial films, interactions between the switched 180° domains and these pre-existing ferroelastic domains dominate the overall polarization-switching kinetics. In particular, the presence of ferroelastic domains reduces the responsiveness of the thin film by lowering the spontaneous out-of-film polarization and reducing the electromechanical piezoelectric response, d 33 , in piezoforce microscopy-switching experiments [1] , [3] . During switching, these domains are often observed to undergo 180° switching in place rather than 90° switching. Although this removes charged domain boundaries between the switched domains and the embedded ferroelastic domains, the polarization is not completely aligned with the applied electric field, leading to the observed decrease in the measured spontaneous polarization. These ferroelastic domains also lead to a decrease in the relative stability of a written domain structure and have been seen to be associated with back switching of the thin film to its initial state after the removal of the applied electric field [3] , [4] . This behaviour is especially important in non-volatile devices as their ability to retain the current state is determined by the stability of newly written domains [5] . Macroscopic ferroelectric-switching studies naturally tend to aggregate interactions between domains into the total system behaviour [6] . An understanding of the local response and underlying dynamic behaviour of individual domain walls and defects throughout the thickness of the film during the switching process is necessary, however, to engineer reliable ferroelectric devices [6] , [7] , [8] , [9] , [10] , [11] , [12] , [13] , [14] . This is especially important in ferroelectric memory devices scaled down to the nanometre scale to achieve a high data storage density where a single defect may dominate the total switching process. At this feature size, it is critical to understand how specific interactions between isolated immobile ferroelastic domains and switched ferroelectric domains influence local switching dynamics. Several studies have attempted to elucidate the specific interactions around ferroelastic domain walls that lead to their strong influence on macroscopic switching kinetics in tetragonal ferroelectrics [2] , [3] , [4] , [15] , [16] . For example, the preferential nucleation of 180° domains at 90° domain walls was reported in barium titanate using optical techniques [15] . Polarization switching through preferential paths was also observed in PZT thin films using piezoresponse force microscopy [3] , whereas numerical modelling of the polarization switching around embedded 90° domains showed that the reduction in the nucleation potential near the domain boundary was the result of a large built-in electrostatic field at the surface of the film lowering the energy barrier to nucleation [17] . The numerical study, however, did not investigate polarization switching beyond the initial nucleation. Ferroelastic domain walls have also been found to be active in switching kinetics beyond facilitating domain nucleation [2] , [4] . Little [15] found, for instance, that in bulk crystals, 180° domain wall motion was abruptly arrested at 90° domain walls. On the basis of electrical measurements, Li and Alexe [2] proposed that 90° domain walls inhibit the motion of 180° domain walls in the plane of the film, slowing the switching kinetics and reducing the overall response of the ferroelectric to an applied electric field. Electrical measurements, however, yield only statistically averaged results, and surface probe techniques are unable to observe subsurface switching paths. Using either method, detailed atomic-scale mechanisms governing the interactions between 90° and 180° domain boundaries are difficult to determine. Understanding local switching pathways, however, is critical as ferroelectrics find use in miniaturized electronic devices such as capacitors and memory devices [9] where the switching kinetics of individual domains dominate the device’s response. To overcome the resolution limits of optical and electrical measurement techniques, we use transmission electron microscopy (TEM) with in situ switching along with numerical phase-field simulations of the full switching process to determine the interaction mechanisms between 90° and 180° domain walls during switching. In comparison with general measurement techniques, in situ TEM can be used to directly observe atomic-scale domain interactions in real time during switching through the thickness of the film, enabling switching dynamics to be correlated with local defect microstructures in real time [13] , [18] , [19] . Employing spherical aberration-corrected TEM with sub-angstrom resolution [20] , [21] , we are able to directly map the local polarization at the atomic scale [9] , [10] . We combine this with mesoscale phase-field modelling of the dynamic polarization-switching processes to corroborate our observations with current models of ferroelectric thin films. Our key finding is the identification of a dipole glass structure formed at the immobile ferroelastic domain boundary during the switching process as the primary atomic-scale mechanism for hindering of the domain-switching process by immobile ferroelastic domains. We find that formation of this layer could occur to reduce the system’s electrostatic energy and allow formation of stable head-to-head domain boundaries in the thin films. The impact of this layer on the switching process and strategies to overcome this effect are discussed. Phase-field modelling Phase-field modelling [22] , [23] , [24] of an isolated 90° domain embedded in a c -poled PZT thin film was used to understand the starting electromechanical state of the film. The results ( Fig. 1a–d ) show that the ferroelastic domain walls develop an electrical charge and are associated with significant strains despite lying on nominally charge and strain neutral {101} planes. In fact, an electrical potential step exists across a ferroelastic domain wall in bulk tetragonal PbTiO 3 according to first-principles calculations [25] and phase-field simulations [26] , indicating 90° domain walls may be inherently charged. In addition, the effect of the substrate constraint may lead to additional polarization charges at the domain wall because of different polarization magnitudes for the c- and a -domains in an epitaxial thin film ( c refers to domains with the polarization oriented along the film normal and a refers to those with the polarization oriented in-plane). The existence of this bound charge can have a significant impact on the local switching dynamics. Because of the presence of charged 90° domain walls, the externally applied bias changes less quickly at the surface of the film, reducing the electric field there ( Fig. 1b,c ). As a result, a larger applied bias is required to generate the critical electric field for switching in the vicinity of the 90° domain wall. In addition, clamping of the ferroelectric film by the epitaxial substrate leads to local inhomogeneous strain distributions ( Fig. 1d ), which may influence local switching kinetics in a more complicated manner. 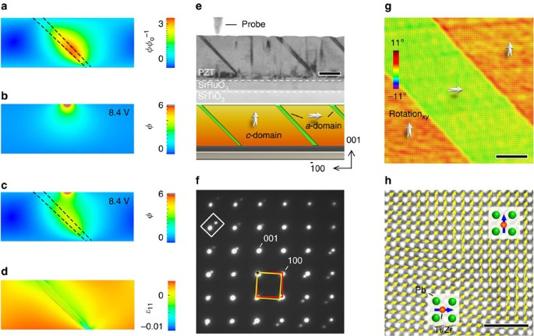Figure 1: Ferroelastic domains in a tetragonal PZT thin film. (a) The calculated potential distribution around an isolateda-domain showing the domain walls are moderately charged. (b) Calculated potential distribution at 8.4 V without and (c) with an embeddeda-domain. (d) Calculated elastic strain distribution in the absence of external bias showing large compressive strain near thea-domain/substrate interface. (e) TEM image of thein situbiasing experimental set-up. A sharp mobile tungsten tip acts as an electrode, whereas the bottom SRO electrode is grounded. Scale bar, 100 nm. The schematic below the micrograph illustrates the observed ferroelastic domains. (f) Selected area electron diffraction pattern acquired from a region including botha-domain andc-domain showing splitting of the diffraction spots. The red rectangle indicates thec-domain diffraction pattern, whereas the yellow rectangle corresponds to thea-domain diffraction pattern. (g) Atomic resolution HAADF image of an embeddeda-domain overlaid with its lattice rotation angle mapping generated by GPA. The colour boundaries correspond to the 90°-domain walls. Scale bar, 5 nm. (h) Plot of polarization vectors for a 90°-domain wall showing head-to-tail configuration. Scale bar, 2 nm. Figure 1: Ferroelastic domains in a tetragonal PZT thin film. ( a ) The calculated potential distribution around an isolated a -domain showing the domain walls are moderately charged. ( b ) Calculated potential distribution at 8.4 V without and ( c ) with an embedded a -domain. ( d ) Calculated elastic strain distribution in the absence of external bias showing large compressive strain near the a -domain/substrate interface. ( e ) TEM image of the in situ biasing experimental set-up. A sharp mobile tungsten tip acts as an electrode, whereas the bottom SRO electrode is grounded. Scale bar, 100 nm. The schematic below the micrograph illustrates the observed ferroelastic domains. ( f ) Selected area electron diffraction pattern acquired from a region including both a -domain and c -domain showing splitting of the diffraction spots. The red rectangle indicates the c -domain diffraction pattern, whereas the yellow rectangle corresponds to the a -domain diffraction pattern. ( g ) Atomic resolution HAADF image of an embedded a -domain overlaid with its lattice rotation angle mapping generated by GPA. The colour boundaries correspond to the 90°-domain walls. Scale bar, 5 nm. ( h ) Plot of polarization vectors for a 90°-domain wall showing head-to-tail configuration. Scale bar, 2 nm. Full size image Ferroelastic domain wall structures Isolated ferroelastic domains were investigated in c -oriented tetragonal PZT films, with a thickness of ~200 nm, grown on {001} SrTiO 3 (STO) substrates buffered with an ~20 nm thick SrRuO 3 (SRO) conducting electrode. Cross-sectional TEM specimens were prepared by conventional mechanical polishing and argon ion milling. A TEM image ( Fig. 1e ) shows a mixture of a / c -domains necessary to accommodate the residual epitaxial stain. A selected area electron diffraction pattern acquired from a region that includes both a -domains (with the polarization oriented towards right) and c -domains (with the polarization oriented upwards) shows the splitting of reflection spots ( Fig. 1f ). There is a lattice tilt, α , of ~2.7° between lattice planes across the 90°-domain wall, corresponding to a lattice constant ratio, c/a = tan (45°+ α /2), of ~1.048, consistent with previous X-ray diffraction results [27] . This lattice tilt enables the 90°-domain walls to be easily distinguished by geometric phase analysis (GPA) [28] of atomic resolution high angle annular dark field (HAADF) images ( Fig. 1g ). Figure 1h shows a map of the polarization vectors around a 90°-domain wall obtained by calculating the offsets of the Pb sublattice [29] , demonstrating that the 90°-domain walls are on {101} planes. This head-to-tail configuration of polarization vectors minimizes the bound charge at the domain wall [7] . This analysis also shows that the width of 90° domain walls is approximately one unit cell according to the polarization vector map in Fig. 1h . In situ ferroelectric switching In situ observations of polarization switching were carried out by application of an electric field between a scanning tungsten tip electrode and the grounded SRO electrode in the TEM ( Fig. 1e ). 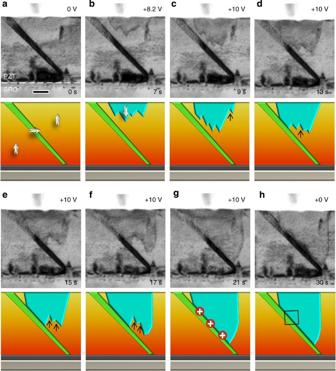Figure 2: Hindering effect of a ferroelastic domain. A chronological TEM bright field image series shows the evolution of a −c-domain at biases of 0→(+10)→0 V. Original polarization ofc-domain in PZT film is upward (a). Scale bar, 100 nm. Nucleation of –c-domain with downward polarization occurs at the top interface of tungsten and PZT at 8.2 V (b). It grows forward slowly with the increase in bias and/or duration (c), but its motion is hindered by the 90°-domain boundary (d–g). After the voltage is removed, the domain is stable with a slight relaxation of the 180°-domain wall (h). Thin arrows indicate possible dislocation pinning sites. Below each image a schematic shows the observed domains. In each image contrast, thermodynamic analysis and high-resolution polarization mapping were used to determine the domain polarization. Figure 2 shows sequential TEM images during switching of a large c -domain adjacent to an a -domain. In Fig. 2b , a new − c -domain (where the negative sign indicates downward polarization) nucleates and grows at the top interface at a bias of 8.2 V, leading to the contrast change from bright to dark. Although previous studies proposed that the nucleation of c -domains preferentially begins from 90° domain walls [3] , [8] , [15] , our in situ TEM observations revealed that nucleation occurs only at the top interface with a negative bias [5] , [10] . The switched − c -domain grew with increasing voltage ( Fig. 2b,c ). Under a constant voltage ( Fig. 2c–g ), the domain grew slowly, which may result from a relatively high density of dislocations acting as weak pinning centres in the film [10] . Dislocations also account for the sawtooth shape of the domain ( Fig. 2c ). As a single needle-like domain was observed in dislocation-free PZT thin films grown on more closely lattice matched DyScO 3 substrates [10] , local pinning causes non-uniform growth of the switched domain front. Figure 2: Hindering effect of a ferroelastic domain. A chronological TEM bright field image series shows the evolution of a − c -domain at biases of 0→(+10)→0 V. Original polarization of c -domain in PZT film is upward ( a ). Scale bar, 100 nm. Nucleation of – c -domain with downward polarization occurs at the top interface of tungsten and PZT at 8.2 V ( b ). It grows forward slowly with the increase in bias and/or duration ( c ), but its motion is hindered by the 90°-domain boundary ( d – g ). After the voltage is removed, the domain is stable with a slight relaxation of the 180°-domain wall ( h ). Thin arrows indicate possible dislocation pinning sites. Below each image a schematic shows the observed domains. In each image contrast, thermodynamic analysis and high-resolution polarization mapping were used to determine the domain polarization. Full size image Once the created − c -domain reached the edge of the a -domain ( Fig. 2d ), the 180°-domain wall motion ceased ( Fig. 2e–g ), showing the ferroelastic domain wall acted as an obstacle to the propagation of the domain wall. When a 180°-domain wall impinges on the ferroelastic domain, the out-of-plane component of the electric field favours the 90°-ferroelastic switching of the a -domain (in which polarization rotates from pointing right to downwards). Such switching, however, is unlikely to happen at moderate field strengths because of the large energy cost associated with the lattice distortion and accompanying elastic strain incurred when switching the ferroelastic domain [30] . In addition, a -domains are often stabilized by misfit dislocations at the film interfaces and consequently are even more difficult to switch [31] , [32] . The pinning observed here differs considerably from that seen in ferroelastic switching in BiFeO 3 by Wrinkler et al. [33] where they observed that growing domains were repelled by pre-existing ferroelastic domain boundaries and that many of these metastable domains disappeared when the bias was removed. In our observations, the switched ferroelectric domain was impeded by the ferroelastic domain and was stable after the removal of applied voltage. Atomically resolved HAADF images were used to characterize the structure of 90° domain walls around the ferroelastic domain after switching ( Fig. 3 ). Mapping the ferroelastic variants around the domain wall using both GPA ( Fig. 3a ) and lattice plane spacing determined from the Pb atom positions ( Fig. 3b ) shows that the lattice orientation change remains sharp across both domain walls during the switching process, and indicates no ferroelastic switching or crystal structure change occurred around the 90°-domain wall during this process. In addition, strain distributions determined from GPA calculations are not obviously affected by the ferroelectric polarization switching ( Supplementary Fig. S1 ). The corresponding polarization angle map calculated by the Pb sublattice offset in Fig. 3c , however, shows that the upper wall is diffuse. There is a transition zone with thickness of ~10 unit cells in which the polarization vectors are randomly oriented and have substantially reduced magnitudes ( Fig. 3e ). As the contrast in a HAADF image comes from the average of many unit cells along the beam direction, it seems that the transition zone consists of many tiny domains polarized in different orientations, resulting in a glassy polarization configuration or dipole glass. Unlike traditional glasses, this region remains crystalline; only the long-range order of the polarization collapses. The uncharged 90° domain wall in the bottom-left corner of Fig. 3c , however, is unaffected and the polarization angle map shows a sharply defined boundary ( Fig. 3f ), similar to that seen before switching ( Fig. 1h ). 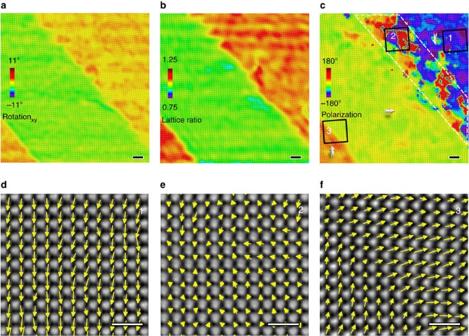Figure 3: Charged ferroelastic domain boundary between −c-domain anda-domain. (a) A map of lattice tilt angle based on GPA calculations overlaid on its atomic resolution HAADF image. The region is the enlarged view of the rectangle inFig. 2h, including three domains: −c-domain (upper right),a-domain (middle) andc-domain (lower left). Scale bar, 2 nm. (b) The map of lattice ratios of out-of-plane to in-plane calculated from the Pb sublattice of the same region. Scale bar, 2 nm. (c) Polarization angle map showing the transition zone, highlighted by the white-dashed line, between −c-domain anda-domain. Scale bar, 2 nm. (d) Polarization vector map of the switcheda-domain corresponding to the rectangle number 1 inc. Scale bar, 1 nm. (e) Polarization vector map from the transition zone corresponding to the rectangle number 2 inc. Scale bar, 1 nm. (f) Polarization vector map at thea-domain/c-domain boundary corresponding to the rectangle number 3 inc. Scale bar, 1 nm. Figure 3: Charged ferroelastic domain boundary between − c -domain and a -domain. ( a ) A map of lattice tilt angle based on GPA calculations overlaid on its atomic resolution HAADF image. The region is the enlarged view of the rectangle in Fig. 2h , including three domains: − c -domain (upper right), a -domain (middle) and c -domain (lower left). Scale bar, 2 nm. ( b ) The map of lattice ratios of out-of-plane to in-plane calculated from the Pb sublattice of the same region. Scale bar, 2 nm. ( c ) Polarization angle map showing the transition zone, highlighted by the white-dashed line, between − c -domain and a -domain. Scale bar, 2 nm. ( d ) Polarization vector map of the switched a -domain corresponding to the rectangle number 1 in c . Scale bar, 1 nm. ( e ) Polarization vector map from the transition zone corresponding to the rectangle number 2 in c . Scale bar, 1 nm. ( f ) Polarization vector map at the a -domain/ c -domain boundary corresponding to the rectangle number 3 in c . Scale bar, 1 nm. Full size image In contrast to previous studies that observed transition layers with suppressed polarization at the substrate interface induced by dislocations [34] , [35] , non-ferroelectric layers at grain boundaries [36] or charge compensation caused irregularly shaped domain walls near the interface [37] ; here the generation of the dipole glass at the charged 90° domain walls may result from the high energy of the head-to-head polarization configuration. As 90° domain walls are on {101} planes, the bound charge density from the termination of the polarization at the domain wall, 2 P S cos θ , is 1.42 P S , where P S is the spontaneous polarization. Given an approximate value for P S of 70 μC cm −2 (ref. 30 ), this corresponds to a charge density of 99 μC cm −2 . Formation of such an energetic, charged domain wall is not favourable, and it is reasonable that a spontaneous relaxation may occur to form a transition zone of mixed polarization to reduce the charge density, increasing the stability of the domain wall. This also reduces the strength of in-plane electric fields at the domain wall that favour 180° ferroelectric switching within the ferroelastic domain such that they are insufficient to cause switching. Therefore, the front of the newly switched − c -domain remains stable and pinned at the a -domain, preventing complete switching at small-to-moderate biases [2] . Such a transition zone only occurs at the charged 90° boundary, whereas the uncharged domain walls remain sharp ( Supplementary Fig. S2 ). With a further increase in applied bias, the transition zone becomes thinner as dipoles in the dipole glass layer are increasingly aligned along the {00-1} direction, leading to an increase in the bound charge density at the boundary. This also increases the in-plane electric field at the boundary and can induce 180° switching within the a -domain, overcoming the hindering effect. 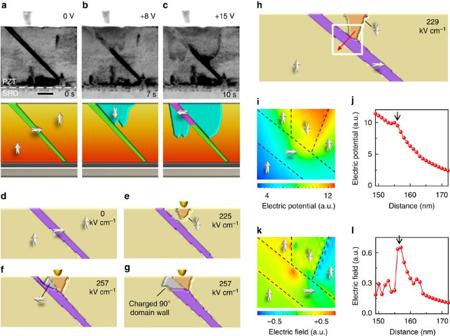Figure 4: One hundred and eighty degree polarization switching within a ferroelastic domain. (a)In situTEM observation of the switching process through an embeddeda-domain. A −c-domain with downward polarization nucleates from the top interface (a,b) at a bias of +8 V, it passes through a ferroelastic domain with the polarization pointing towards right (c) at a bias of approximately +15 V and keeps growing at +15 V. (c) Polarization rotation (180°) has occurred within the ferroelastic domain. Below each TEM image a schematic shows the domain orientations determined using a combination of image contrast, thermodynamic analysis and high-resolution polarization mapping. Scale bar, 50 nm. (d) Phase-field simulation of the switching process around an embeddeda-domain. The switched −c-domain (e) nucleates directly underneath the electrode and extends into the film. Near the charged 90°-domain wall, large in-plane electric fields cause the nucleation of a switched −a-domain with the polarization pointing towards left (f). Thea-domain is replaced by an −a-domain, creating another charged 90° domain wall, which facilitates the switching of farc-domain with upward polarization (g). (h) Simulation of the switched −c-domain impeded by ana-domain at an averaged field of ~229 kV cm−1. (i) The local distribution of electric potential of the rectangle region inh. (j) The potential profile along the red arrow inh. The thin black arrow indicates the location of the charged domain wall. (k) The local distribution of the in-plane electric field of the rectangular region inhindicating large in-plane fields across the charged boundary. (l) The in-plane electric field profile along the red arrow inh. The thin black arrow indicates the charged domain wall. Figure 4a–c shows that at +15 V, the a -domain is switched into a − a -domain (with the polarization pointing left), allowing the 180°-domain wall to pass through the a -domain and continue to grow forward ( Fig. 4b,c ). Although the 180°-domain wall in the a -domain is not shown clearly in Fig. 4c , we did observe it in other cases, as shown in Supplementary Fig. S3 . In addition, if the polarization within the a -domain had not switched, the upper and lower 90° domain walls would become oppositely charged, inducing a large electric field within the a -domain that would favour 180° switching [4] . Figure 4: One hundred and eighty degree polarization switching within a ferroelastic domain. ( a ) In situ TEM observation of the switching process through an embedded a -domain. A − c -domain with downward polarization nucleates from the top interface ( a , b ) at a bias of +8 V, it passes through a ferroelastic domain with the polarization pointing towards right ( c ) at a bias of approximately +15 V and keeps growing at +15 V. ( c ) Polarization rotation (180°) has occurred within the ferroelastic domain. Below each TEM image a schematic shows the domain orientations determined using a combination of image contrast, thermodynamic analysis and high-resolution polarization mapping. Scale bar, 50 nm. ( d ) Phase-field simulation of the switching process around an embedded a -domain. The switched − c -domain ( e ) nucleates directly underneath the electrode and extends into the film. Near the charged 90°-domain wall, large in-plane electric fields cause the nucleation of a switched − a -domain with the polarization pointing towards left ( f ). The a -domain is replaced by an − a -domain, creating another charged 90° domain wall, which facilitates the switching of far c -domain with upward polarization ( g ). ( h ) Simulation of the switched − c -domain impeded by an a -domain at an averaged field of ~229 kV cm −1 . ( i ) The local distribution of electric potential of the rectangle region in h . ( j ) The potential profile along the red arrow in h . The thin black arrow indicates the location of the charged domain wall. ( k ) The local distribution of the in-plane electric field of the rectangular region in h indicating large in-plane fields across the charged boundary. ( l ) The in-plane electric field profile along the red arrow in h . The thin black arrow indicates the charged domain wall. Full size image As the switching process within the a -domain is usually too fast and local to observe with in situ TEM, the phase-field modelling technique [22] , [23] , [24] was employed to simulate the switching around an embedded a -domain and reveal the detailed dynamics. In agreement with the experimental results, the simulation reproduced the hindering effect and 180° switching of the embedded 90° domain boundary during the switching process. Figure 4d–g shows that the progression of domain growth during the simulation is similar to the experimental observations. Initially, the switched − c -domain nucleates directly underneath the electrode and extends into the thin film ( Fig. 4d,e ). The simulation results in Fig. 4h–l show that the interaction between the bound charges at the a -domain wall and the switched − c -domain wall generates a large depolarization potential and in-plane electric field. These fields subsequently lead to the nucleation of 180° switching within a -domains to reduce the bound charge in the region between the a -domain and the switched − c -domain ( Fig. 4f ). Under continued applied potential, this switched − a -domain replaced the previous a -domain, forming another, charged, head-to-head 90° domain wall with the far c -domain ( Fig. 4g ), which facilitates the 180° switching in the far c -domain. Incomplete switching caused by pre-existing ferroelastic domain wall pinning may account for the degraded performance in ferroelectric devices operating at low fields [1] , [2] . Our in situ TEM studies demonstrate that the hindering effect of 90° ferroelastic domains on 180° ferroelectric switching can be overcome by applying higher electric bias ( Fig. 4 ). This is consistent with previous reports on the enhancement of ferroelectric response by improving the mobility of the as-grown a -domains with high-electric field pulses [16] or using nanofabricated island structures [1] . Reversing the applied voltage, the recently created domain can be switched back, as shown in Fig. 5 . The back switching is typically realized by shrinking of the c -domains due to the bound charges at the domain walls, essentially exactly reversing the domain growth process ( Fig. 5a–d ). Eventually, the film returns back to the original domain structure ( Fig. 5d ). The negative voltage required for back switching is smaller than the positive switching voltage because of the built-in electrical field induced by the Schottky barrier between PZT and SRO, which favours the upward polarization and hence facilitates back switching [10] . 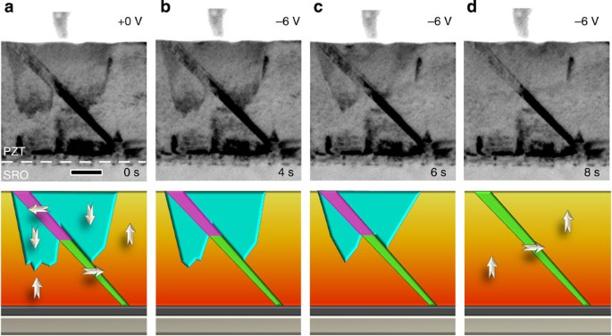Figure 5: Back switching. Reversing the voltage, the switched domain shrinks (a–c), passing through the ferroelastic domain (d) as a result of back switching. Simultaneously, the whole ferroelastic domain is switched back to original state ind. Below each TEM image a schematic shows the domain orientations determined using a combination of image contrast, thermodynamic analysis and high-resolution polarization mapping. Scale bar, 50 nm. Figure 5: Back switching. Reversing the voltage, the switched domain shrinks ( a – c ), passing through the ferroelastic domain ( d ) as a result of back switching. Simultaneously, the whole ferroelastic domain is switched back to original state in d . Below each TEM image a schematic shows the domain orientations determined using a combination of image contrast, thermodynamic analysis and high-resolution polarization mapping. Scale bar, 50 nm. Full size image In conclusion, our results clearly show that ferroelastic a -domains in tetragonal PZT thin films hinder motion of ferroelectric 180° domain walls by forming charged ferroelastic domain boundaries, leading to incomplete switching. To the best of our knowledge, the atomic-scale structure of these charged 90° domain wall is observed for the first time in this study. Charged 90° domain walls exhibit ‘smearing’ of the local polarization at the interface and a ‘dipole glass’ transition layer formed by introducing nanodomains consisting of reduced polarization and disorder to reduce the charge density and depolarization energy, while the charged and uncharged 180° domain wall ( Supplementary Fig. S3 ) and uncharged 90° domain walls ( Fig. 1h ) remain sharp. We propose that the formation of this layer provides the fundamental atomic-scale mechanism for hindering at ferroelastic walls during switching, preventing a simpler, lower voltage-switching process through ferroelastic domains in PZT. This mechanism also probably explains similar hindering at ferroelastic domain walls observed in other ferroelectrics such as rhombohedral BiFeO 3 (ref. 13 ). This result also indicates that a charged 90° domain wall may have an even larger energy density than that of a charged 180° domain wall because of the charge–strain coupling. Material synthesis and characterization Epitaxial PZT and SRO films were grown on single crystal {001} STO substrates by 90 o off-axis sputtering [38] . SRO was grown at 560 °C and 200 mTorr with 3:2 ratio of Ar to O 2 and PZT was grown at 530 °C and 200 mTorr with a 1:1 ratio of Ar to O 2 gasses. Cross-sectional TEM samples were made by conventional mechanical polishing and argon ion milling (Gatan). Atomic resolution scanning TEM images used in this manuscript were acquired using the FEI Titan 80-300 (TEAM 0.5) at Lawrence Berkeley National Lab. In situ TEM In situ TEM experiments were carried out with a JEOL 2010F and a spherical aberration ( C s )-corrected JEOL2100F using a Nanofactory TEM-scanning tunnelling microscopy platform. Electrical bias was applied between a home-made tungsten tip, acting as a movable electrode, and the conductive SRO bottom electrode, which was connected to ground. External voltages were applied using a HP 6614c for direct current voltages and a HP 3324a function generator for triangle waveforms. The domain evolution was recorded by a (Gatan) charge-coupled device or a (Gatan) television-rate camera at 29 frames using diffraction contrast imaging with diffraction g =202 p . Phase-field modelling Phase-field modelling is a mesoscale-modelling approach that evolves the distribution of the three polarization components, P i , in time towards a minimum energy state by solving the time-dependent Ginzburg–Landau equation [22] , [23] , [39] , [40] , [41] In equation (1), F is the volume integral of the total free energy of the system expressed in terms of the polarization components and L is the kinetic coefficient. The phase-field model considers contributions to the total free energy from the bulk free energy, f bulk ; the electrical dipole interaction energy, f electric ; the elastic interaction energy, f elastic ; and the polarization gradient energy, f gradient . Altogether, the total free energy expressed in terms of the polarization parameters has the form [39] , [40] where f i are the local contributions of each type of energy. In equation (2), the strain distribution is introduced as a second-order parameter to model the elastic response of the system [23] . Bulk crystal free energy was modelled using a sixth-order Landau polynomial of the form: where α 1 , α 11 , α 12 , α 111 , α 112 and α 123 are the empirical fitting parameters for the Landau polynomial to describe phase transitions in Pb(Zr 0.2 Ti 0.8 )O 3 under stress-free conditions. For this simulation, coefficients measured by Haun, et al. [42] , [43] , [44] were used. Electrical dipole interactions between bound polarization charges and the electric field distribution, E i , were considered through the electrostatic interaction energy [24] , [45] In equation (4), ε 0 is the permittivity of free space and κ ij is the relative background dielectric constant tensor. Using a specified polarization distribution, the electric field distribution was found by first finding the potential distribution, ϕ , through the Poisson equation [24] and using this result to determine the electric field via E i =− ϕ ,i . For the thin film geometry with an electrically conductive bottom electrode under an applied bias, fixed electrical potential boundary conditions at the film surfaces were used to solve equation (5). For the planar bottom electrode in the system, the potential was held uniformly constant at zero bias throughout the simulation. In contrast, the electrode used at the top surface for switching was modelled using a piezoresponse force microscope (PFM)-like potential simulated using the Lorentz-like distribution of width γ (ref. 17 ) In equation (6), the centre of the electrode potential distribution was assumed to be located at position ( x 0 , y 0 ) and to apply a potential, ϕ 0 , at the centre of the distribution. For these simulations, the applied potential distribution width parameter γ was assumed to have a value of 10 nm. Ferroelectric PZT undergoes a spontaneous deformation, ε ij 0 , as a result of the electrostrictive effect. Elastic energy associated with the resulting total strain in the system, ε ij , is (ref. 23 ) where C ijkl is the stiffness tensor of PZT. The spontaneous strain associated with the ferroelectric transformation in equation (6) is related to the polarization via the experimentally measured electrostrictive tensor, Q ijkl Similar to the potential, the strain distribution was determined for a given polarization distribution by solving the equations for mechanical stability in the thin film: Details about solving equations (7, 8, 9) for the film/substrate system and the required boundary conditions are presented in depth elsewhere [23] , [39] . Domain wall energy in the system was included through the polarization gradient energy. For the sake of simplicity, isotropic gradient energy was assumed, so the total gradient energy was expressed as (ref. 23 ) In equation (10), G 1111 is the gradient energy coefficient. For this simulation, its value was chosen to be G 1111 / G 110 =0.6 in reduced units. G 110 was related to the voxel size in the simulation Δ, through . For an assumed grid spacing of Δ=1 nm, G 110 =1.5 × 10 −10 C −2 m 4 N. Using equations (3, 4, 5, 6, 7, 8, 9, 10), the temporal evolution of the thin film under an applied potential was obtained by using a linear approximation to the time derivative in equation (1) and solving the resulting equation using the semi-implicit Fourier spectral method [22] . This method applies periodic boundary conditions in the x 1 and x 2 dimensions while applying the specified boundary conditions in the out-of-plane x 3 dimension. For this simulation, a regular grid of 256Δ × 48Δ × 96Δ voxels was used with periodic boundary conditions along the first two dimensions. The thickness of the film was taken to be 56Δ while the substrate was assumed to have a thickness of 14Δ (ref. 39 ). Each cubic voxel was assumed to have an edge length of 1 nm. Further, the substrate was assumed to apply a biaxial substrate strain to the film of –0.7% as a result of the lattice mismatch between the STO substrate and Pb(Zr 0.2 Ti 0.8 )O 3 film. This strain represents a partially relaxed biaxial strain in the system and was applied by assuming a constant average background strain when solving equation (9) above. Several layers of substrate were included to allow some small relaxation of the substrate in response to deformation in the film. However, for solving equation (9), the displacement at the bottom of the substrate was assumed to be zero. The time step used was Δ t =0.01 where Δ t =1/( L | α 1 | T =25 °C ) (ref. 23 ). In Fig. 1a–c , the potential distribution is normalized by a characteristic potential defined in the simulation as ( HP 0 | α 11 | T =25 °C ) where H is the voxel edge length and P 0 is the spontaneous polarization assumed to be around 0.757 Cm −2 . In all, the characteristic potential is 0.123 V. How to cite this article: Gao, P. et al. Atomic-scale mechanisms of ferroelastic domain-wall-mediated ferroelectric switching. Nat. Commun. 4:2791 doi: 10.1038/ncomms3791 (2013).